Robust self-cleaning and micromanipulation capabilities of gecko spatulae and their bio-mimics Geckos have the extraordinary ability to prevent their sticky feet from fouling while running on dusty walls and ceilings. Understanding gecko adhesion and self-cleaning mechanisms is essential for elucidating animal behaviours and rationally designing gecko-inspired devices. Here we report a unique self-cleaning mechanism possessed by the nano-pads of gecko spatulae. The difference between the velocity-dependent particle-wall adhesion and the velocity-independent spatula-particle dynamic response leads to a robust self-cleaning capability, allowing geckos to efficiently dislodge dirt during their locomotion. Emulating this natural design, we fabricate artificial spatulae and micromanipulators that show similar effects, and that provide a new way to manipulate micro-objects. By simply tuning the pull-off velocity, our gecko-inspired micromanipulators, made of synthetic microfibers with graphene-decorated micro-pads, can easily pick up, transport, and drop-off microparticles for precise assembling. This work should open the door to the development of novel self-cleaning adhesives, smart surfaces, microelectromechanical systems, biomedical devices, and more. Many organisms rely on sophisticated micro-/nano-fibrillar structures, patterns and/or textures to obtain intricate surfaces with optimized multifunctionality. Some prominent examples include lotus leaves [1] , spider silks [2] , shark skins [3] , butterfly scales [4] and fish-hair flow sensors [5] . Of particular interest is the hierarchically structured toe pads of geckos, which enable the animals to climb and dance on wet or dry, smooth or rough, clean or dusty, vertical or even inverted surfaces with ease [6] . Though very ‘sticky,’ gecko feet remain extremely clean for periods of months between moulting cycles [7] . Our recent experimental results demonstrate that after its feet are contaminated, a live gecko sheds dirt from its toes, returning its feet to about 80% of its original stickiness in only four steps [8] . Such extraordinary self-cleaning ability stems from the hierarchical structures of gecko toes, consisting of millions of micro-fibrils, called setae ( Fig. 1a,b,f ); these branches further split into hundreds to thousands of nano-sized platelet-shaped pads, called spatulae ( ∼ 10 nm thick and ∼ 200 nm wide; inset of Fig. 1c ) [9] , [10] . Mimicking these hierarchical fibrillar adhesive structures, one can create a new generation of sticky, yet self-cleaning materials for various applications, such as reusable tapes, climbing robots, smart and switchable surfaces, and biomedical devices, to name a few. Various synthetic gecko adhesives have been fabricated using silicones, urethanes, plastics, carbon nanotubes and other materials, to generate adhesive forces up to 10 times stronger than that of the gecko foot [11] , [12] , [13] , [14] . Despite these successes, synthetic reusable adhesives with self-cleaning capabilities comparable to those of the gecko adhesives have not yet been obtained. The fact is that the self-cleaning ability is a major factor in keeping gecko feet reliably sticky over time; even adhesive tapes, no matter how sticky they are, become useless as they pick up dirt. Therefore, to successfully translate the self-cleaning capabilities of gecko adhesives into bio-inspired adhesives, it is necessary to gain an understanding of the fundamental principles governing the self-cleaning process in gecko adhesion. 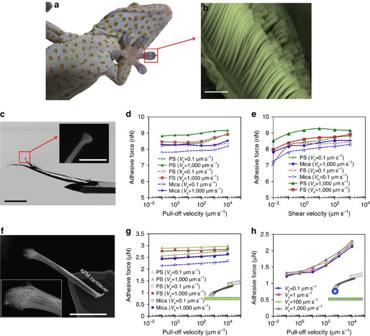Figure 1: Structure and dynamic adhesive force of gecko setae and spatulae. (a) Optical image of a gecko sole. SEM images of (b) setal array (scale bar, 20 μm) and (c) a single spatula (isolated from a seta) glued onto a tipless AFM cantilever (scale bar, 20 μm; inset, 500 nm). Adhesive forces of the single spatula on mica, FS and PS substrates versus (d) pull-off velocity (Vn) and (e) shear velocity (Vs) for a preload of 10 nN and a drag distance of 4 μm. (f) SEM images of a single seta glued on a tipless AFM cantilever(scale bar, 30 μm). (g) Adhesive forces of the single seta on mica, FS and PS substrates as a function of the pull-off velocity at given shear velocities ofVs=0.1 and 1,000 μm s−1for a preload of 1 μN, and a drag distance of 4 μm (inset: the schematic of a single seta in making contact with a substrate). (h) Adhesive forces of a SiO2microsphere (diameter,d=10 μm) adhered to a seta as a function of the pull-off velocity for a preload of 1 μN and a drag distance of 1 μm (inset: the schematic of microsphere-seta complex, in making contact with fused silica substrate). All the tests are performed in air with a relative humidity of 21% at room temperature. Figure 1: Structure and dynamic adhesive force of gecko setae and spatulae. ( a ) Optical image of a gecko sole. SEM images of ( b ) setal array (scale bar, 20 μm) and ( c ) a single spatula (isolated from a seta) glued onto a tipless AFM cantilever (scale bar, 20 μm; inset, 500 nm). Adhesive forces of the single spatula on mica, FS and PS substrates versus ( d ) pull-off velocity ( V n ) and ( e ) shear velocity ( V s ) for a preload of 10 nN and a drag distance of 4 μm. ( f ) SEM images of a single seta glued on a tipless AFM cantilever(scale bar, 30 μm). ( g ) Adhesive forces of the single seta on mica, FS and PS substrates as a function of the pull-off velocity at given shear velocities of V s =0.1 and 1,000 μm s −1 for a preload of 1 μN, and a drag distance of 4 μm (inset: the schematic of a single seta in making contact with a substrate). ( h ) Adhesive forces of a SiO 2 microsphere (diameter, d =10 μm) adhered to a seta as a function of the pull-off velocity for a preload of 1 μN and a drag distance of 1 μm (inset: the schematic of microsphere-seta complex, in making contact with fused silica substrate). All the tests are performed in air with a relative humidity of 21% at room temperature. Full size image To date, a few possible self-cleaning mechanisms have been proposed, including: (i) ultra-hydrophobic surfaces that resist unwanted adhesion [15] , (ii) the lotus effect [1] , (iii) ultra-hydrophilic surfaces [16] and (iv) contact with unbalanced normal forces and shear drag [7] , [17] , [18] , [19] , [20] , [21] . As the first three mechanisms involve the action of water, they cannot explain the dry self-cleaning associated with the gecko’s sticky footpads. The contact mechanism can explain how dirt particles are dislodged from the adhesives, but it is unclear why the self-cleaning rate of a live gecko is much higher than that of manipulated setal arrays [7] , [8] . Since gecko walking is a dynamic process involving contact/separation of gecko setae/spatulae with dirt particles and/or surfaces, their dynamic effect may play a key role in promoting self-cleaning of gecko adhesive systems. Some dynamic phenomena, such as frictional adhesion, have been observed in gecko and synthetic adhesives [22] , [23] , [24] , [25] , [26] , and the theory has been applied to explain the phenomena [27] , [28] . However, knowledge of the potential role of the dynamic effect of setae and spatular nano-pads in the entire self-cleaning process is very limited. In this study, we investigate the adhesion and self-cleaning responses when dynamic processes are applied on fundamental nanoscale elements in gecko adhesive systems, namely the spatular pads, during dynamic release of gecko feet under both wet and dry conditions. We find that gecko spatulae and setae have distinctive dynamic behaviours compared with dust/sphere particles, providing critical design principles for the development of robust self-cleaning systems. We also create a biomimetic micromanipulator, based on the rational concepts of spatula dynamics. Dynamic effects of single seta and spatula at the nanoscale Using an atomic force microscope (AFM), we examine the dynamic adhesion of an individual spatula on a variety of substrates in customized chamber environments. A single spatula specimen is made with a focused ion beam (FIB) by removing all but one spatular branch from a single seta that is glued on the back of a tipless AFM cantilever ( Fig. 1c ). Mimicking the natural motions of gecko feet (that is, subjecting the spatula to a load–drag–pull constraint [29] , [30] , as schematically illustrated in Supplementary Fig. 1 ), the spatula is brought into contact with the substrates, followed by a proximally directed shear drag with a drag distance, s , at a shear velocity of V s , and then a 90° pull-off at a normal velocity of V n . This procedure allows us to record dynamic adhesive forces when the AFM cantilever is pulled off the substrates at given speeds ( V n ) in the normal direction, during a shear drag at given shear velocity V s . Notably, this loading process also simulates the footpad hyperextension during gecko walking, which will be discussed in details in the following sections. In comparison, adhesive forces of the individual seta ( Fig. 1f ) and a microparticle that is firmly adhered to a seta (inset of Fig. 1h ) are also measured with the same procedure. Note that the shear and normal (pull-off) velocities measured here are those applied on the setal roots that are glued on the AFM cantilevers. The typical force-time curve for a seta on a mica substrate during the load–drag–pull procedure and the force-displacement curves for the spatulae, setae and microparticles are shown in Supplementary Fig. 2a,b,c and d , respectively. As observed in our previous experiments [29] , [31] , strongly normal-velocity-dependent adhesion occurs when a microsphere is pulled off from various substrates in normal directions both in air and under water ( Supplementary Fig. 3 ). By contrast, the spatulae show weakly normal-velocity-dependent adhesive forces with a large variety of substrates, including polystyrene (PS), mica, and fused silica (FS), over a wide range of pull-off velocities, from 0.01 to 20,000 μm s −1 ( Fig. 1d ). In contrast to the weakly-dependent effects of increasing pull-off velocity, increasing the shear velocity enhances the adhesion ( Fig. 1e ). Other factors such as drag distance, contact time and humidity also enhance the adhesion ( Supplementary Figs 4 and 5 ). To further verify if the dynamic effect of the pull-off also occurs in synthetic mimics, and is therefore not an inherently material-based phenomenon, we fabricate a spatula-shaped platelet ( ∼ 500 nm in size; Supplementary Fig. 11a,b ) at the end of glass microfibers (10 μm in diameter) via FIB. These nano-crafted microfibers are then tested on the AFM using the same set-up and procedures as used in the spatula pull-off experiments. Similar to gecko spatulae, the nano-platelet terminated artificial fibrils exhibit almost invariant adhesive strengths with increasing velocity ( Supplementary Fig. 11c ). Thus, the dynamic effects of the spatular platelet are distinctive and duplicable. Similar normal-velocity-independent phenomenon is also observed for single setae. The adhesive force is nearly independent of pull-off velocity but enhanced by increasing the shear velocity ( Fig. 1g , and Supplementary Fig. 6 ), drag distance, contact time ( Supplementary Fig. 7a,b ) and humidity ( Supplementary Fig. 8 ). Furthermore, the adhesive forces of single seta on various substrates, including microparticles ( Supplementary Fig. 9 ) and plant leaves ( Supplementary Fig. 10a ), are measured under water and in air with different humidities and contact times. Once again, the nearly normal-velocity-independent adhesion holds in all cases. The effects of the humidity and contact time can be attributed to the condensation of water from ambient air into the gap just outside the periphery of the contact interface (or water bridging), which introduces capillary forces, ultimately resulting in an increase in the measured pull-off force. This condensation occurs only if at least one of the solids (the spatula/seta, the particle or the surface) is hydrophilic [30] . Since the spatula and seta are highly hydrophobic materials [32] , their adhesive forces are less sensitive to the pull-off velocity and humidity variations. As shown in Supplementary Fig. 8 , the adhesive forces of setae on teflon, a typical hydrophobic surface, are less sensitive to humidity variations than other substrates. Interestingly, it is also observed that the adhesive forces of setae on plant leaves are strong both in air and under water, whereas other substrates (for example, mica) show relatively weak adhesion under water ( Supplementary Fig. 10a ); this explains why geckos living in rain forests can generate sufficient adhesion on wet leaves [32] . Unlike the clean setae that show normal-velocity-independent adhesive forces, a ‘contaminated’ seta (that is, the seta firmly adhered with a microparticle at its tip, as schematically shown in the inset of Fig. 1h ) exhibits a normal-velocity-dependent behaviour on various substrates ( Fig. 1h ), including the plant leaves ( Supplementary Fig. 10b ). Because the pristine spatulae and setae show normal-velocity-insensitive adhesion, whereas ‘dirt’ particles adhered onto setae result in normal-velocity-sensitive dynamic adhesion, we hypothesize that the tip shape of spatulae may be the direct cause of strong resistance to the unwanted dirt particles during setal release, perfectly combining the self-cleaning with strong adhesion and easy detachment of gecko’s feet over a wide range of environments. Dynamic self-cleaning mechanism and manipulation of setae It is well known that before taking each step during animal locomotion, most geckos hyperextend their toes to disengage their feet by peeling the toe pads from distal to proximal directions [8] , [33] . During the digital hyperextension, individual setae are sequentially pulled off from the substrates at relatively high speeds, as schematically shown in Fig. 2a . Each seta undergoes a normal pull-off displacement Δ y , as well as a lateral displacement Δ x at its root, before its tip completely detaches from substrate. Using a scrolling model [8] , we can calculate the lateral and normal displacements as Δ x = r [ ωt −sin( ωt )] and Δ y = r [1−cos( ωt )], and the resultant retreating velocities of the setal root as V s = ωr [1−cos( ωt )] in lateral (shear) direction, and V n = ωr sin( ωt ) in normal direction, respectively, where r is the scrolling radius of the toe pad, t is time, and ω is the rotational angular velocity of the toe pad. Taking the pull-off distance Δy ∼ 1.5 μm from the seta pull-off experiment ( Supplementary Fig. 2c ), r =3,000 μm, and ω =125–315 rad s −1 , (ref. 8 ) we estimate V n =10,000–30,000 μm s −1 . During the pull-off process, the hyperextension also generates shear velocity (that is, V s =170–450 μm s −1 , assuming no macro slipping effect) from distal to proximal sides, but it is minimal compared with normal velocity. Note that these velocities of setae induced by the digital hyperextension are conceptually different from the gecko running speed (0.29–0.77 m s −1 ; ref. 34 ), because the animal running speed (that is, body speed) is generated by the forward thrust from the engaged feet through its limbs, whereas the speed at the setal roots is generated by hyperextension during engaged stage when the feet keep stationary relative to the ground. Although the hyperextension-induced speed of setal roots is relatively low compared with the gecko running speed, it is high enough to cause the particle-substrate adhesive force ( F w-p ) to overcome the seta-particle adhesive force ( F s-p ), resulting in effective self-cleaning. 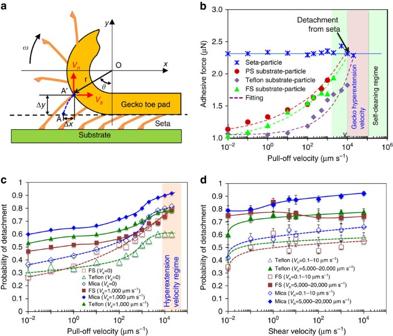Figure 2: Gecko hyperextension and the probability of particle detachment from single setae. (a) Schematic of gecko toe pad scrolling motion under digital hyperextension, which is modelled as a rolling motion of a circle, with a radiusr, along a horizontal plane. The trajectory of a setal root (for example, from point A to A’) follows the corresponding cycloid curve (for example, blue dashed line) depending on the specific location of each seta. The hyperextension generates normal velocity (Vn) as well as shear velocity (Vs) on the setal roots. (b) Dynamic adhesion responses between single seta and glass microsphere (Fs-p) and those between SiO2microparticles (d=10 μm) and FS, PS and teflon substrates (Fw-p) with increasing pull-off velocity (Vn). Probability of the SiO2particle (d=10–15 μm) detachment events from setae in 30-time trials on fused silica, mica and Teflon substrates as a function of (c) the pull-off velocity for shear velocities of 0, and 1,000 μm s−1and a preload of 1 μN, and (d) shear velocity at a preload of 1 μN for different pull-off velocities (error bar: s.d.). For the seta-particle contact experiments in (b), the microparticles are detached from the seta at 1,000–10,000 μm s−1, depending on the type of substrates. These values are critical velocitiesVc, above which the particles are detached from the setae. Note that the pull-off velocity of gecko setae during animal walking is estimated to be 10,000–30,000 μm s−1, larger than the critical velocityVc, suggesting that Tokay geckos’ adhesive toe pads are always in the ‘self-cleaning regime’ during animal locomotion. The estimated gecko pull-off velocity is illustrated in (b) and (c). Figure 2: Gecko hyperextension and the probability of particle detachment from single setae. ( a ) Schematic of gecko toe pad scrolling motion under digital hyperextension, which is modelled as a rolling motion of a circle, with a radius r , along a horizontal plane. The trajectory of a setal root (for example, from point A to A’) follows the corresponding cycloid curve (for example, blue dashed line) depending on the specific location of each seta. The hyperextension generates normal velocity ( V n ) as well as shear velocity ( V s ) on the setal roots. ( b ) Dynamic adhesion responses between single seta and glass microsphere ( F s-p ) and those between SiO 2 microparticles ( d =10 μm) and FS, PS and teflon substrates ( F w-p ) with increasing pull-off velocity ( V n ). Probability of the SiO 2 particle ( d =10–15 μm) detachment events from setae in 30-time trials on fused silica, mica and Teflon substrates as a function of ( c ) the pull-off velocity for shear velocities of 0, and 1,000 μm s −1 and a preload of 1 μN, and ( d ) shear velocity at a preload of 1 μN for different pull-off velocities (error bar: s.d.). For the seta-particle contact experiments in ( b ), the microparticles are detached from the seta at 1,000–10,000 μm s −1 , depending on the type of substrates. These values are critical velocities V c , above which the particles are detached from the setae. Note that the pull-off velocity of gecko setae during animal walking is estimated to be 10,000–30,000 μm s −1 , larger than the critical velocity V c , suggesting that Tokay geckos’ adhesive toe pads are always in the ‘self-cleaning regime’ during animal locomotion. The estimated gecko pull-off velocity is illustrated in ( b ) and ( c ). Full size image To verify this self-cleaning mechanism, we measure the adhesive forces F w-p and F s-p for various microparticles under identical testing conditions. When pulling off a seta that is in contact with a particle on a substrate, we would have two scenarios for the particle: either drop off (Case I) or pick up (Case II) by the seta, as schematically shown in Supplementary Fig. 12d . In Case I, the particle is dropped off from the seta if it binds more strongly to the substrate than to the seta ( F w-p > F s-p ); conversely, in Case II, the particle is picked up by the seta when it binds more strongly to the seta than to the substrate ( F w-p < F s-p ). In Case I, the seta remains clean naturally, but in Case II, it is contaminated by the particles. Figure 2b shows a case (Case II), in which F w-p is estimated to be two times smaller than F s-p at a low speed of V n <1 μm s −1 . In this case, the microparticles on the substrates are successfully picked up by the seta. With increasing V n , F w-p increases and eventually surpasses F s-p at a critical point V c , (for example, V c ∼ 2,000 μm s −1 for a 10-μm SiO 2 particle on PS substrate), leading to the detachment of the particle from the seta. Thus, self-cleaning occurs at high pull-off velocities even if the adhesive force of the seta to the particle is initially stronger than that of the particle to the substrate. For the first time, this dynamic self-cleaning mechanism has been directly observed at the microscopic level ( Supplementary Movie 1 , a particle is picked up from a surface at a low normal velocity (for example, ∼ 10 μm s −1 ); Supplementary Movie 2 , the attached particle is dropped off on the surface at a high normal velocity (for example, ∼ 1,000 μm s −1 ) for a shear velocity of 100 μm s −1 and a drag distance of 5 μm). It should be noted that the pull-off velocity induced by hyperextension (gecko hyperextension velocity) is higher than these critical values V c , indicating that gecko setae are always in a ‘self-cleaning regime’ during gecko locomotion, as illustrated in Fig. 2b . To correlate the nanoscale dynamic phenomenon to the self-cleaning ability at the gecko foot level, we mimic gecko walking via AFM to manipulate a single seta to repeatedly approach and contact particles on a substrate, drag a distance ( s ) horizontally, and then retreat normally from the substrate, as schematically shown in Supplementary Fig. 12 . The probability of the particle drop-off (detachment) events (that is, Case I in Supplementary Fig. 12d ) in a 30-trial is obtained for different pull-off velocities, shear velocities, drag distances and preloads, and plotted in Fig. 2c,d and Supplementary Figs 13 and 14 , respectively. The average probability of particle detachment is about 40% for fused silica, PS and mica substrates at a low velocity of V n =0.1 μm s −1 , but it rapidly ramps up with increasing the pull-off velocity and reaches 80% at V n =20,000 μm s −1 ( Fig. 2c ). Surprisingly, the values of the probability are almost identical to those of the force recovery indexes measured ( ∼ 40% for no hyperextension, and ∼ 80% for hyperextension) in our previous experiment at the whole animal scale of live geckos [8] . A plausible explanation is that the force recovery index is directly correlated with the amount of dirt shed from the gecko feet (or setal arrays) [8] , and the probability is a measure of the tendency of the dirt to detach from the gecko seta, the two of which are directly correlated. Thus, the distinctive dynamic force effects of spatulae and setae identified at the micro-/nanoscale are closely related to the self-cleaning ability observed at the macroscale. To the best of our knowledge, such a self-cleaning effect, achieved by tuning pull-off velocity, is a new phenomenon observed at the micro- and macro-levels. It is worth noting that the dynamic effect is also very strong at the nanoscale in both dry and aqueous environments ( Supplementary Fig. 3 ), allowing nanoparticles to be cleaned via the same mechanism in different environments. As shown in Fig. 2d and Supplementary Fig. 13 , increasing the shear velocity and drag distance also increases the detachment probability (that is, self-cleaning), but this influence levels off beyond the critical values (for example, ∼ 10 μm s −1 for the shear velocity, and ∼ 2 μm for the drag distance). This increase in the probability can be attributed to the change in seta-particle interface states, induced by the shear drag. Although the particle is still adhered to the seta after the dragging, the seta-particle contact interface is already changed by the dragging through mechanisms, including breaking of the possible water bridge, interfacial bonding, and/or spatula contact points. Since the particles are pre-adhered, dragging can alter the seta-sphere interface more significantly than the sphere-substrate one (fresh contact), thus increasing the detachment probability. When a seta with a pre-adhered particle is dragged over a longer distance (for example, over 10 μm), we observe that the adhered particles could be sheared off the seta, resulting in self-cleaning. This pure shear drag or rolling-induced self-cleaning phenomenon has been observed in gecko and synthetic adhesive systems [17] , [18] , [19] , [20] , [21] . However, if only the shear drag is applied, the particles that are detached from setae by the shearing/rolling effects could reattach to other setae in setal arrays during the gecko foot sliding. In contrast to the shearing, the normal pull-off action induced by hyperextension provides a possibility for all the particles that strongly adhere to the setae to dislodge from the setae at the same time, which is a more robust and efficient self-cleaning process. Despite not being a dominating factor, the shear velocity enhances the dynamic effect during normal pull-off, and consequently the self-cleaning efficiency. Dynamic self-cleaning of biomimetic micromanipulator Inspired by the unique spatular structure and its dynamic effect, we fabricate artificial setae using synthetic polyester microfibers (10 μm in diameter). Each fibre (150 μm in length) is cut to form a micro-pad at its tip, then bonded to an AFM cantilever ( Fig. 3a ). This is followed by a layer-by-layer gluing of three layers of wrinkled graphene multilayers ( ∼ 5 nm thick) on the micro-pad ( Fig. 3b,c , Supplementary Figs 15 and 16 ). The use of graphene layers can drastically enhance the adhesion capability of the artificial setae, as graphene has been previously reported to generate ultra-strong adhesion over various surfaces [35] . The wrinkled graphene layers on a pad, mimicking gecko spatulae on a seta, could also increase the surface compliance and contact area to further enhance the adhesion. Unlike traditional adhesives (for example, Scotch tape), the graphene layer can generate reversible/tunable adhesion, which is critical to a variety of applications, including self-cleaning and small object manipulation in air and under water. Using the artificial seta attached on an AFM probe as a micromanipulator, we successfully manipulate microspheres on various substrates, and are able to pick up, translate and precisely assemble the micro-sized particles ( d =1–20 μm) in a patterned fashion ( Fig. 3d ). The manipulation processes are demonstrated (pick up at low pull-off speed, Supplementary Movie 3 , and drop off at high pull-off speed, Supplementary Movie 4 ). In addition to microspheres, the micromanipulator can also manipulate other types of small objects, such as debris and microfiber segments ( Supplementary Movie 5 ). 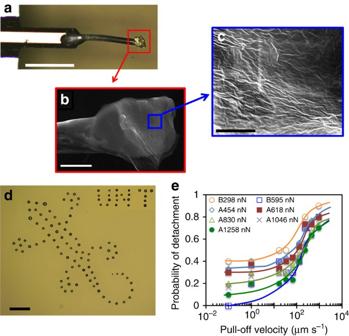Figure 3: Micromanipulation of microparticles by artificial setae. (a) Optical image of the biomimetic micromanipulator made of a polyester microfiber (d=10 μm,L=150 μm) with a graphene layer-decorated micro-pad at its tip, glued on an AFM tipless cantilever (front view). (b) SEM image of the micro-pad with three layers of (c) wrinkled graphene (thickness:∼5 nm) on the top. (d) Optical image of a gecko pattern and a logo precisely assembled with SiO2microparticles (size:d=1–25 μm) on a glass slide by the biomimetic micromanipulator. (e) Probability of particle detachment as a function of pull-off velocity, measured with 30-trials, mimicking gecko walking (shear velocityVs=4 μm s−1, drag distances=2 μm, and contact timetc=0). A and B in the legend refer to two micromanipulators A and B, and the numbers are values of preloads. Scale bar in a–d: 100, 10, 5, and 100 μm, respectively. Figure 3e shows the probability of microsphere detachment events in a 30-trial experiment. Similar to the natural setae, the probability of particle detachment is within a range of 0–40% at low pull-off velocity, but rapidly ramps up and reaches ∼ 80% at a normal pull-off velocity of ∼ 1,000 μm s −1 . Figure 3: Micromanipulation of microparticles by artificial setae. ( a ) Optical image of the biomimetic micromanipulator made of a polyester microfiber ( d =10 μm, L =150 μm) with a graphene layer-decorated micro-pad at its tip, glued on an AFM tipless cantilever (front view). ( b ) SEM image of the micro-pad with three layers of ( c ) wrinkled graphene (thickness: ∼ 5 nm) on the top. ( d ) Optical image of a gecko pattern and a logo precisely assembled with SiO 2 microparticles (size: d =1–25 μm) on a glass slide by the biomimetic micromanipulator. ( e ) Probability of particle detachment as a function of pull-off velocity, measured with 30-trials, mimicking gecko walking (shear velocity V s =4 μm s −1 , drag distance s =2 μm, and contact time t c =0). A and B in the legend refer to two micromanipulators A and B, and the numbers are values of preloads. Scale bar in a–d: 100, 10, 5, and 100 μm, respectively. Full size image It is desirable that the micromanipulator can reliably and repetitively pick up and drop-off particles or other small objects. As can be seen from Fig. 3d and Supplementary Fig. 17 , the detachment probability is almost zero at a low speed of V n <1 μm s −1 and a relatively high preload of 1.3 μN, suggesting that the micromanipulator can pick up the particles with nearly 100% success. In contrast, at high pull-off speed ( V n ∼ 1,000 μm s −1 ) and low preload ( ∼ 0.4 μN), the probability is close to one, indicating that the micromanipulator can reliably drop-off particles. Apart from the pull-off velocity and preload force, the shear velocity also affects the probability. Similarly to the natural setae, increasing the shear velocity increases the detachment probability of the micromanipulator, but its effect quickly reaches a plateau ( Supplementary Fig. 18 ), suggesting that the shear velocity is important but not a dominating parameter in the manipulation process. To examine the durability of the biomimetic micromanipulator, we repeatedly make the attachment and detachment on a glass substrate at a frequency of 1 Hz and a preload of 1 μN, and found no abnormality even after 100,000 cycles. In case the pads are damaged, the micromanipulator can be feasibly repaired by gluing a new layer of graphene on these pads, indicating strong reusability. These results demonstrate that the self-cleaning and micromanipulation capabilities based on the distinctive dynamic effect of gecko spatular nano-pads are robust and efficient in synthetic bio-inspired adhesives as well. Modelling dynamic effects of spatulae setae and particles A multiscale modelling approach is developed to gain more insight into the distinctive dynamic effects of gecko spatula and seta, which are responsible for the dynamic self-cleaning ability and micromanipulation mechanism. At the nanoscale, a finite element model with a cohesive zone is developed to simulate the pull-off process of spatulae after the shear drag is made ( Fig. 4a , Supplementary Fig. 19 ). The cohesive elements are built between the spatula pad and a rigid substrate to simulate adhesion and separation along the interface ( Supplementary Note 1 ). At the microscale, a seta consisting of 256 spatular branches ( Fig. 4e , Supplementary Fig. 21 ) is built based on the hierarchical setal structure [36] , and simulations are carried out to predict its dynamic behaviour during the pull-off process ( Supplementary Note 3 ). The force-displacement relationship obtained from the spatula simulation is input into the upper-scale seta simulation to represent spatula–substrate interactions. In comparison, a finite element model with a similar cohesive zone along the particle-substrate interface is also developed to simulate the pull-off process of microspheres on a substrate ( Fig. 4c , Supplementary Fig. 20 and Supplementary Note 2 ). The properties of spatula, seta and microsphere, and their cohesive zones are listed in Supplementary Table 1 . In the pull-off simulations, displacements in the normal direction at given velocities ( V n ) are exerted on the ends of the spatular and setal shafts, and the particle top. The adhesive forces are determined based on the maximum values of the force-displacement curves. 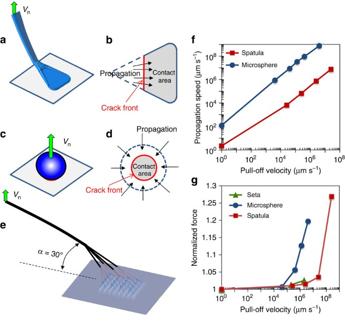Figure 4: Multiscale modelling of dynamic adhesion of single seta single spatula and microsphere. Schematics of pulling (a) a single spatula and (c) a microparticle from a flat substrate, corresponding to two distinctive mechanisms of crack propagation along (b) the spatula/substrate interface (that is, the advancing crack front line increases in length from the vertex to tip-edge), and (d) the microsphere/substrate interface (that is, the advancing crack front circle reduces in length in radial direction), respectively. (e) Finite element analysis (FEA) models for a single seta with 256 spatular branches in pull-off simulations, (f) Average crack propagation velocity (Vp) as a function of pull-off velocity (Vn), predicted by the FEA simulation, and (g) Adhesive forces of the microsphere (d=10 μm), single spatula and single seta, normalized by their adhesive forces at the static state, predicted by the FEA models, as a function of pull-off velocity. Figure 4: Multiscale modelling of dynamic adhesion of single seta single spatula and microsphere. Schematics of pulling ( a ) a single spatula and ( c ) a microparticle from a flat substrate, corresponding to two distinctive mechanisms of crack propagation along ( b ) the spatula/substrate interface (that is, the advancing crack front line increases in length from the vertex to tip-edge), and ( d ) the microsphere/substrate interface (that is, the advancing crack front circle reduces in length in radial direction), respectively. ( e ) Finite element analysis (FEA) models for a single seta with 256 spatular branches in pull-off simulations, ( f ) Average crack propagation velocity ( V p ) as a function of pull-off velocity ( V n ), predicted by the FEA simulation, and ( g ) Adhesive forces of the microsphere ( d =10 μm), single spatula and single seta, normalized by their adhesive forces at the static state, predicted by the FEA models, as a function of pull-off velocity. Full size image The separations of the spatula and the microsphere from their substrates during the pull-off stages can be considered as crack propagation processes along the spatula-substrate and sphere-substrate interfaces, respectively. However, because of their distinctive interfacial configurations, the spatula exhibits a completely different propagation behaviour from the microsphere—this difference in propagation schemes has important implications on adhesive forces. When a spatula is properly engaged onto a flat substrate, a triangle-shaped contact area forms and the possible crack propagation is constrained in the direction from the vertex to the front edge as the spatula is retracted [37] , [38] . Under these conditions, the crack propagates in a constrained manner, since the crack front line has to increase while it advances ( Fig. 4b ). Similar crack-like propagation is observed in the seta pull-off simulation. The seta pull-off induces unidirectional crack propagation process along the distributed interfaces from proximal to distal directions ( Supplementary Fig. 22 ). In contrast, for a microsphere being pulled off from a flat substrate, the crack growth is considerably ‘unstable’, because the crack front line (that is, a closed circular or loop, Fig. 4d ) rapidly decreases in length during the separation process. This unstable configuration results in much higher crack propagation speeds along the interface. We calculate the average crack propagation speed ( u ) against the pull-off velocity ( V n ) for a spatula on a rigid surface and a 10-μm SiO 2 microsphere adhering on a flat glass substrate ( Fig. 4f ). The average propagation speeds for both the spatula and the particle increase nearly linearly with increasing pull-off velocity, but at a given V n , the spatula has a propagation speed nearly three orders of magnitude lower than that of the particle. It is well known in fracture mechanics that there are several regimes of behaviour in crack propagation. According to the Griffith energy balance concept, in a quasistatic regime the energy release rate G is roughly constant and equal to a material dependent critical energy release rate, G c (ref. 39 ). In unstable configurations, or during fast loading, however, the kinetic energy becomes important, leading to a dynamic regime [40] . The dynamic effects may originate from the energy dissipations (for example, internal friction and viscous effects) at the interface between the particle and surface. In general, G is directly correlated to the propagation speed u by a power law relationship [41] : G = G 0 [1+( u / u 0 ) m ], where G 0 is the critical energy release rate as u is approaching zero, m is a scaling parameter that is empirically fitted to the experimental data, and u 0 is the crack propagation speed at which G doubles to G 0 . Since G can be further related to the interfacial adhesive force, the crack propagation speed (or pull-off velocity) can be linked to the adhesive forces [29] , [31] . From above analysis, it concludes that the relatively low propagation speed at the spatula-substrate interface would significantly reduce the dependence of the adhesive force on the pull-off velocity. We calculate the adhesive forces at different pull-off velocities for the seta, the spatula and the microsphere ( Fig. 4g ). There is a significant difference in dynamic behaviour between the spatula and the microsphere. While the adhesive force for microspheres rapidly increases after V n >1,000 μm s −1 , the significant increase for spatulae and setae occurs after V n >1,000,000 μm s −1 ( Fig. 4g ), indicating that the spatular geometry is more tolerant than spherical contact when subjected to dynamic external loadings, in terms of the crack propagation shift from quasistatic to dynamic regimes. These simulation results explain well the experimental results that the adhesive forces of the spatulae and setae are much less sensitive to the pull-off velocity variations in the range 0–1,000,000 μm s −1 , and provide insight behind the experimental results. Hansen and Autumn suggested the contact self-cleaning mechanism, in which self-cleaning occurs when F w-p > F s-p (ref. 7 ). In other words, small solid particles may bind more strongly to the substrate than to the toe pads. Consequently, when pressing a contaminated toe pad against a clean surface multiple times, the particles are removed from the toe pads via a force imbalance. Interestingly, their results show ∼ 40% force recovery for gecko setal arrays when simulating gecko walking [7] , the value of which is almost the same as the results of our probability experiments at the low pull-off velocity regime ( Fig. 2c ). However, for those particles that bind more strongly to the toe pads than to the substrate surface, that is, F w-p < F s-p , according to the contact self-cleaning mechanism [7] , self-cleaning cannot take place at quasistatic states (low pull-off speeds). In our experiment, we show that even if F w-p < F s-p , at the quasistatic state, self-cleaning can still occur at high pull-off velocities ( Fig. 2c ). This newly identified dynamic self-cleaning mechanism increases the efficiency of the self-cleaning by a factor of 2, compared with that reported by Autumn and others [7] , [20] . In fact, it is found in our previous experiment that a live gecko sheds dirt from its toes, recovering nearly 80% of its original stickiness in only four steps [8] . This whole animal experiment is consistent with our results for a single seta tests under dynamic loadings (that is, probability of particle detachment: ∼ 80% at high pull-off speed). This proposed dynamic self-cleaning mechanism, stemming from the distinctive dynamic contact characteristics of spatula, explains the higher self-cleaning rate of live geckos very well [8] . In addition, our results show that the shear velocity also plays a role in enhancing the self-cleaning efficiency. During animal locomotion, active digital hyperextension generates high normal pull-off speed as well as shearing speed before each step, effectively and efficiently dislodging the dirt from its toes in a progressive manner, which keeps the gecko’s feet sticky yet clean. In summary, this study has provided direct evidence that the unique shape of nanoscale spatula pads plays a crucial role in generating robust and stable adhesion while permitting efficient self-cleaning capabilities in dynamic regimes. Furthermore, emulating the gecko self-cleaning principle has led to the design of novel artificial setae as powerful micromanipulation tools, which can viably manipulate and precisely assemble micro-/nano-particles by tuning pull-off velocity. It is foreseeable that this self-cleaning mechanism has important impacts on the development of many biologically inspired technologies, including smart and antifouling surfaces, micro-/nano-assemblies, under water cell manipulation technologies, and microelectromechanical systems devices. Preparation of single seta and spatula of geckos Setal arrays are collected from live Tokay geckos and immediately stored in a sealed container to prevent contamination from dust and moisture. Newly unpackaged glass slides are cleaned in deionized water with an ultrasonic cleaner (Ultrasonic cleaner 1510, Branson Co., Inc.) for 15 min, then dried out in air before tests. First, individual setae are carefully collected from the intact setal arrays under an optical microscope with a micromanipulator (Mode 2525, The Micromanipulator Co. Inc.) and placed onto the cleaned glass slides. Operated by an atomic force microscope (AFM) micromanipulator system (Scan-Icon AFM, Bruker Co., Inc.), a tipless cantilever (ACTA-TL-50, AppNano) is then maneuvered to capture a tiny glue droplet (diameter ∼ 10 μm), placed on the same glass slide, at the underside of its free end, then translated toward a nearby target gecko seta, and finally pressed onto the root portion of the seta for permanent bonding. A 30-min slow cure epoxy (Kite studio Co., Inc.) is used as the glue to make sure there is sufficient time for the entire bonding procedure to take place before the adhesive hardens. Since natural setae have a particular orientation on gecko toe pads, only those setae glued at the base, such that the spatula branches are flushing downwards at the free end, are cured for measurements. The glued setae are cured in air at room temperature for 24 h, then examined under an optical microscope to make sure that their orientation is correct before subsequent experiments. After tests, the setae glued onto the AFM cantilevers are carefully examined by a scanning electronic microscope (FEI Quanta ESEM) to determine their length, diameter and orientation. To prepare individual spatulae for adhesion measurement, a FIB (Dual Beam FIB/FESEM FEM Nova 200) is used to remove all but one spatular branch from a single seta that is glued on the backside of a tipless AFM cantilever, such that only a single spatular pad is in contact with the substrate surface. Low voltage is crucial to prevent the electron beam from damaging the integrity of the setae/spatulae. Preparation of artificial spatula and micromanipulators The artificial spatulae are also fabricated using the FIB system. Glass microfibers with a length of 140 μm and a diameter of 10 μm are pre-glued at the free end of tipless AFM cantilevers with the method described above. The fibre tips are then crafted into spatula-like geometries. For preparation of the biomimetic micromanipulators, polyester fibres (diameter: 10 μm) are cut with scissors, and then the fibre segments (length: 150 μm) with a naturally cut pad at one end are selected and pre-glued to AFM cantilevers. A piece of clean monolayer graphene synthesized by chemical vapour deposition [42] is selected and glued to the pad of the microfibers using the 30-min slow cure epoxy. To make the pad softer, three layers of graphene are glued to the pad after 24 h curing by repeating the procedure above. More layers could be glued to the pad to repair damage during use. This makes the biomimetic micromanipulators reusable. Measurement of adhesive force in air or under water A variety of flat target substrates with different hydrophobicities/hydrophilicities are employed, including glass, mica, sapphire, FS, PS and teflon, all of which are AFM sample kits from Bruker, CA, USA, with surface roughnesses of <5 nm. The attachment and detachment of individual gecko setae/spatulae from the substrates is operated by the ‘closed-loop’ AFM system, mimicking gecko walking (that is, setae subjected to a load–drag–pull constraint [29] , [30] ). As schematically shown in Supplementary Fig. 1 , the AFM cantilever movement is controlled to approach a surface or a microsphere, make contact, then horizontally move at a controlled shear speed in the range of 0.1 ∼ 10 4 μm s −1 , and finally retreat at a controlled pull-off speed in the range of 10 −2 ∼ 10 5 μm s −1 . The interaction force and displacement of the AFM (z-piezo) are recorded during each test. The spring constant of each AFM probe is measured with a thermal tune method and the average spring constant is obtained to be ∼ 40 N m −1 . To measure the adhesive forces between seta/spatula and substrates under water, a drop of ∼ 200 μl of deionized water is applied onto the substrates, and an AFM cantilever glued with setae, spatulae or microparticles is then completely immersed into the drop. The adhesive force is measured in the same procedure as in air. When tested in water, in addition to the particle–substrate interaction force, the AFM cantilever itself is also subject to a hydrodynamic effect (for example, drag) due to the movement of the cantilevers. This water drag resistance to the cantilevers is measured by moving the cantilevers in water at different speeds. The dynamic effect of the cantilever due to the drag can then be removed from the forces measured in the pull-off test. Therefore, the adhesive forces posted in this paper are the particle–substrate interaction forces only. More details of operations in air and water can be found elsewhere [29] , [31] . Measurement of adhesive force between setae and particles Microparticles made of polystyrene, SiO 2 and Al 2 O 3 , with average diameters of 10 μm (C-Ps −1 0.0, C-SIO-10.0, and C-ALU-10.0, Microsphere-Nanosphere Inc.), are used as the fouling agents. These particles are cleaned using the same procedure used on the flat substrates, and the resultant colloidal partial-water dispersions are then applied onto a clean glass slide and dried at room temperature for 24 h. Then, the dried particles are transferred to another clean glass slide by tapping the dirtied glass slide over the new slide to form a randomly distributed single particle layer, mimicking a naturally dusted area. During AFM pull-off tests at a given velocity, in some cases a microsphere can adhere ‘firmly’ to a fresh setal tip to form a microsphere-seta complex, and the forces obtained are recorded as occurring between particle and wall, F w-p ; in the cases where a microsphere is not picked up by the setal tip during retraction, the measured adhesive force represents the interaction force between the setae and microparticles ( F s-p ). Modelling dynamic effects of spatulae setae and particles A three-dimensional finite element model of a single gecko spatula is developed to simulate the dynamic effect of spatula. The model consists of a nano-platelet, a shaft, rims and a spatula-substrate contact interface. The spatula-substrate interface is treated as a cohesive layer with three-dimensional cohesive elements. A traction-separation law [43] is used for the cohesive elements to simulate the crack initiation and evolution process. An axisymmetric finite element model of a microsphere in contact with a substrate is also developed to simulate the particle pull-off experiment. The model consists of a microsphere, a substrate and an interface. Similar to the spatula model, the microsphere-substrate interface is treated as a cohesive layer with cohesive elements. The same traction-separation law is used for the cohesive elements to simulate the crack initiation and evolution process. A finite element model for a single gecko seta is also created to simulate the adhesive force during seta retraction from substrates at different pull-off velocities. The setal shaft and branches are modelled by one-dimensional beam elements, while the spatula-substrate contact interface is described by three-dimensional cohesive elements. The pull-off simulations of the spatulae, setae and microspheres are performed using the commercial finite element package, Abaqus/Explicit (6.10). How to cite this article: Xu, Q. et al . Robust self-cleaning and micromanipulation capabilities of gecko spatulae and their bio-mimics. Nat. Commun. 6:8949 doi: 10.1038/ncomms9949 (2015).